B7-H5 costimulates human T cells via CD28H The B7/CD28 family has profound modulatory effects in immune responses and constitutes an important target for the development of novel therapeutic drugs against human diseases. Here we describe a new CD28 homologue (CD28H) that has unique functions in the regulation of the human immune response and is absent in mice. CD28H is constitutively expressed on all naive T cells. Repetitive antigenic exposure, however, induces a complete loss of CD28H on many T cells, and CD28H negative T cells have a phenotype of terminal differentiation and senescence. After extensive screening in a receptor array, a B7-like molecule, B7 homologue 5 (B7-H5), was identified as a specific ligand for CD28H. B7-H5 is constitutively found in macrophages and could be induced on dendritic cells. The B7-H5/CD28H interaction selectively costimulates human T-cell growth and cytokine production via an AKT-dependent signalling cascade. Our study identifies a novel costimulatory pathway regulating human T-cell responses. Current research supports the notion that T-cell activation and tolerance are orchestrated by the co-signalling network [1] , [2] , [3] . The B7/CD28 family molecules have critical and unique roles among co-signalling molecules, and the B7/CD28 axis was the first to be identified and the most extensively studied ligand/receptor complex for T-cell costimulation [4] , [5] , [6] . Among its various effects on T cells, CD28 has been recognized as a major costimulatory receptor specialized in priming pan naive T cells, and promoting both T-cell division and cytokine production, especially interleukin 2 (IL-2) in secondary lymphoid organs [7] . CD28 signalling prevents T-cell anergy, the unresponsiveness status of T cells to antigen challenge [8] , [9] . Moreover, survival of activated T cells can be enhanced by CD28 costimulation, in part by the upregulation of the survival factor, Bcl-xL [10] . CTLA-4, the counterpart for CD28, is critical for the maintenance of T-cell tolerance, because disruption of its interaction with B7-1 and B7-2 leads to broad and profound lymphocyte infiltration in the peripheral and lymphoid organs [7] . The important role of the B7/CD28 family in the modulation of immune response has been highlighted by three biologics drugs approved by the FDA and several promising agents in clinical trials for the treatment of human diseases. Infusion of CTLA4-Fc recombinant fusion protein Abatacept or Belatacept has been shown to be beneficial for the patients with rheumatoid arthritis or kidney transplantation rejection, respectively [11] , [12] . Ipilimumab (Yervoy), a CTLA-4 monoclonal antibody (mAb) with the capacity to block its coinhibitory function, systemically activates T cells, which leads to enhanced antitumour immunity and therefore a survival benefit in 10–15% patients with advanced metastatic melanoma [13] . More recently, a phase I/II trial of PD-1 mAb demonstrated an objective clinical response in ~1/3 of the patients with advanced non-small-cell lung cancer, kidney cancer and melanoma with minimal toxicity [14] , [15] , [16] . In this study, we describe a new receptor–ligand interaction in the B7/CD28 family, between CD28H and B7 homologue 5 (B7-H5). CD28H is constitutively expressed on naive T cells while its ligand B7-H5 is found broadly in professional antigen-presenting cells (APCs) and in peripheral organs. The interaction of B7-H5/CD28H has profound costimulatory functions in human T-cell responses both in vitro and in vivo . As this interaction is absent in mice, our findings warrant reassessment of the knowledge obtained from mouse models of lymphocyte co-signalling. Identification and characterization of CD28H An extensive genome-wide search was performed to identify genes that are both preferentially expressed on T cells and homologous to CD28. Through this search, we discovered a new human gene previously called transmembrane and immunoglobulin domain containing 2 (gene ID 126259). No function has been designated for this gene. Therefore, we renamed it CD28 homologue (CD28H) to reflect its close relationship with CD28. The human CD28H gene locates on chromosome 19q13.3, and it consists of five exons and spans about 10.2 kb ( Fig. 1a ). The CD28H gene encodes a putative single transmembrane protein, which is composed of a single immunoglobulin variable-like (IgV) domain, one transmembrane domain and a long intracellular domain ( Fig. 1b ). Alignment of the amino-acid sequence of CD28H to other CD28 family members indicates that CD28H shares over 10% identity with CD28, CTLA, ICOS and PD-1 ( Supplementary Fig. S1a ). Phylogenic tree analysis further reveals that CD28H is closer to CD28 than PD-1 in amino-acid similarity ( Fig. 1c ). CD28H seems to be conserved in zebra fish, guinea pig, cow and chimpanzee, because all these species have CD28H orthologs and inferred protein-coding sequences ( Supplementary Fig. S1b ). However, mouse and rat do not have the coding gene for CD28H, although there are traces of CD28H gene fragments present in their genomes. 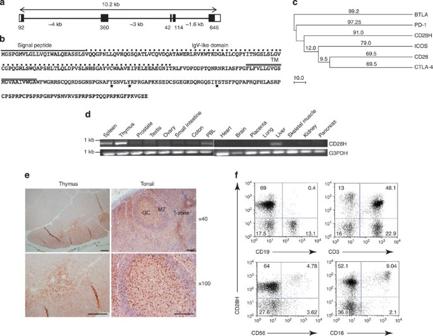Figure 1: Characterization of human CD28H. (a) Genomic organization of humanCD28Hgene. Each box represents an exon which is separated by an intron with indicated length. Filled boxes indicate coding sequences in exons, and unfilled boxes indicate the 3'- and 5'-untranslated regions. The number of nuclear acids in each exon is indicated below. (b) Protein sequence encoded by the humanCD28Hgene. Predicted signal peptide, IgV-like, and transmembrane domains with three tyrosines are indicated. (c) Guide tree analysis of human CD28H and the known CD28 family members via Clustal W program in MacVector 6.5. (d) PCR analysis of human CD28H transcript using human multiple cDNA panels from Clontech. (e) Immunostaining of CD28H in human thymus and tonsil tissues (Scale bar, 100 μm). (f) Flow cytometry analysis of CD28H expression on human PBMCs from healthy donors stained with indicated cell surface markers. Figure 1: Characterization of human CD28H. ( a ) Genomic organization of human CD28H gene. Each box represents an exon which is separated by an intron with indicated length. Filled boxes indicate coding sequences in exons, and unfilled boxes indicate the 3'- and 5'-untranslated regions. The number of nuclear acids in each exon is indicated below. ( b ) Protein sequence encoded by the human CD28H gene. Predicted signal peptide, IgV-like, and transmembrane domains with three tyrosines are indicated. ( c ) Guide tree analysis of human CD28H and the known CD28 family members via Clustal W program in MacVector 6.5. ( d ) PCR analysis of human CD28H transcript using human multiple cDNA panels from Clontech. ( e ) Immunostaining of CD28H in human thymus and tonsil tissues (Scale bar, 100 μm). ( f ) Flow cytometry analysis of CD28H expression on human PBMCs from healthy donors stained with indicated cell surface markers. Full size image PCR analysis of human tissue complementary DNAs indicated that the CD28H transcript was preferentially enriched in lymphoid organs ( Fig. 1d ). The thymus and spleen had the highest levels of CD28H messenger RNA (mRNA). In addition, peripheral blood lymphocyte (PBL) and liver also contained abundant CD28H transcript. We generated a mAb against human CD28H. The specificity of CD28H mAb was verified by its binding to CD28H transfectants, but not HEK293T cells transfected with other CD28 family members ( Supplementary Fig. S2a ). Thymus and tonsil tissues contained a significant number of cells that stained positive for CD28H ( Fig. 1e ). Most immature CD4-CD8− double-negative thymocytes did not express surface CD28H. However, thymocytes in the CD4+CD8+ double-positive stage were CD28H+, as were the CD4+ or CD8+ single-positive cells in the thymus ( Supplementary Fig. S3 ). We also analysed CD28H expression in the peripheral blood mononuclear cells (PBMCs) of healthy human donors using flow cytometry. No detectable surface CD28H was found on B cells. The majority of natural killer (NK) cells, defined as CD56+ or CD16+ cells, constitutively expressed high levels of CD28H. Similarly, a large portion of CD3+ T cells from the PBMCs of the healthy donors constitutively expressed CD28H ( Fig. 1f ). T-cell activation leads to loss of CD28H Further examination of CD28H expression on adult human T-cell subsets by flow cytometry revealed that both CD4+ and CD8+ αβT-cell subsets contained a similar percentage of T cells constitutively expressing CD28H ( Fig. 2a ). In contrast, virtually all γδT cells were CD28H−. Virtually all T cells from human cord blood, presumably naïve T cells, expressed high levels of CD28H ( Supplementary Fig. S4 ). We further examined CD28H expression on subsets of human CD8+ T cells based on CCR7 and CD45RA expression [17] . All naive T cells (Tn, CD45RA+CCR7+) constitutively expressed CD28H ( Fig. 2b ). About half the T cells with central memory (CD45RA−CCR7+) and effector memory (CD45RA−CCR7−) phenotypes were CD28H+. The majority of CD45RA+ effector memory (T EMRA ) cells (CD45RA+CCR7−), presumably terminally differentiated effector T cells, loss their CD28H expression [17] , [18] . Similar findings were observed in CD4+ T-cell subsets ( Supplementary Fig. S5a ). CD28H− T cells purified from PBMCs did not contain CD28H transcript, suggesting that CD28H expression on T cells is controlled in transcription level ( Supplementary Fig. S5b ). We further stained T cells for CD28H expression together with various T-cell surface markers. CD28H− T cells were higher in side scatter, and most of them expressed CD45RO but not CD45RA ( Supplementary Fig. S5c ). In addition, the expression of activation-induced molecules such as PD-1 was increased whereas the levels of CD62L and CD27 were reduced in CD28H− cells [19] , [20] . Consistently, the CD28H− T cells comprised the population prone to the secretion of effector cytokines and lytic molecules upon activation ( Supplementary Fig. S5d ). Similarly, most effector cytokine-producing CD4+ T helper cells or FoxP3+ CD4+ T regulatory (T reg ) cells did not express CD28H ( Supplementary Fig. S5e ). 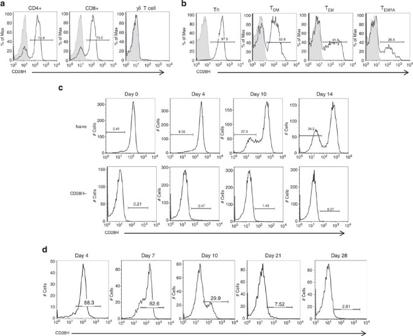Figure 2: Regulation of CD28H expression in human T cells. (a) CD28H expression on CD4+CD3+, CD8+CD3+ and γδT-cell subsets. (b) CD28H expression on different CD8+ T-cell subset. CD8+ T cells were stained with anti-CD45RA, anti- CCR7 and anti-CD28H mAbs. Upon analysis of CD45RA and CCR7 expression, four subsets of CD8+ T cells were identified: Tn(CD45RA+CCR7+), TCM(CD45RA−CCR7+), TEM(CD45RA−CCR7−) and TEMRA(CD45RA+CCR7−). Numbers indicate percentages of CD28H+ cells in each population. Data are from three independent experiments (one representative of three donors). (c) Regulation of CD28H expression on T cells upon T-cell division. Purified naive or CD28H− human T cells were fully activated by OKT3 together with anti-CD28 mAb and recombinant human IL-2. Ten days after culture, living cells were collected and restimulated under the same conditions. The expression of CD28H on T cells was indicated at different time points by flow cytometry. (d) CD28H expression upon T-cell proliferationin vivo. Naïve human CD4+ T cells were transferred into NSG mice. The expression of CD28H on transferred T cells was analysed on the indicated dates. Figure 2: Regulation of CD28H expression in human T cells. ( a ) CD28H expression on CD4+CD3+, CD8+CD3+ and γδT-cell subsets. ( b ) CD28H expression on different CD8+ T-cell subset. CD8+ T cells were stained with anti-CD45RA, anti- CCR7 and anti-CD28H mAbs. Upon analysis of CD45RA and CCR7 expression, four subsets of CD8+ T cells were identified: T n (CD45RA+CCR7+), T CM (CD45RA−CCR7+), T EM (CD45RA−CCR7−) and T EMRA (CD45RA+CCR7−). Numbers indicate percentages of CD28H+ cells in each population. Data are from three independent experiments (one representative of three donors). ( c ) Regulation of CD28H expression on T cells upon T-cell division. Purified naive or CD28H− human T cells were fully activated by OKT3 together with anti-CD28 mAb and recombinant human IL-2. Ten days after culture, living cells were collected and restimulated under the same conditions. The expression of CD28H on T cells was indicated at different time points by flow cytometry. ( d ) CD28H expression upon T-cell proliferation in vivo . Naïve human CD4+ T cells were transferred into NSG mice. The expression of CD28H on transferred T cells was analysed on the indicated dates. Full size image One possible cause of the loss of CD28H expression on antigen-experienced T cells is repetitive antigen stimulation. To test this, we purified naive (virtually all CD28H+) or CD28H− T cells from fresh PBMCs, and stimulated them with anti-CD3 plus anti-CD28 in the presence of IL-2. Full T-cell activation was achieved in 4 days, as demonstrated by the high levels of CD69 expression and the loss of CD62L. CD28H+ T cells maintained 100% of their CD28H expression throughout 4 days’ culture ( Supplementary Fig. S6a and Fig. 2c ). Activated T cells were rested for 3 days and restimulated on day 7. A small population of T cells started to lose CD28H on day 10. On day 14 the CD28H− T-cell population increased to 34% ( Fig. 2c ). In addition, CD28H mRNA was not detectable on those newly generated CD28H− T cells ( Supplementary Fig. S6b ). On the other hand, when CD28H− T cells were activated, none of those T cells gained CD28H expression during the 14-day period of stimulation. Together, these results suggest that repetitive stimulations induce the irreversible loss of CD28H expression on naive T cells. The loss of CD28H on T cells upon cell activation was also confirmed in vivo . When naive human T cells were transferred into immunodeficient NOD- SCID Il2rg −/− (NSG) mice, human T cells proliferated vigorously responding to xenogeneic antigens in mice [21] accompanied with progressive loss of CD28H: T cells started to lose CD28H on day 7 and more than half of the transferred human T cells had lost CD28H on day 10 and nearly all T cells were CD28H− on day 28 ( Fig. 2d ). Persistent immune activation causes loss of CD28 expression in human T cells, which represent a group of later-stage differentiated T cells [22] . We costained human CD8+ T cells with CD28H and various surface molecules, which are associated with human T-cell senescence [23] , [24] , [25] , [26] . Almost all T cells with senescent phenotype (CD7lowCD27−CD28−CD57+) were exclusively CD28H− ( Supplementary Fig. S7a ). We labelled purified CD28H+ naive and CD28H− T cells with carboxyfluorescein diacetate succinimidyl ester (CFSE), and assessed their proliferative capacity to T-cell antigen receptor (TCR) signalling. Though CD28H+ naive T cells proliferate vigorously, virtually no cell division was detected in CD28H− T cells in response to the same concentration of anti-CD3 ( Supplementary Fig. S7b ). To exclude the possibility that the slower division of CD28H− T cells is caused by a small population of internal suppressive T cells (for instance, FoxP3+ T reg cells Supplementary Fig. S5e ), we labelled whole PBMCs with CFSE and tested their response to anti-CD3 within 7 day, when the majority of T cells do not change CD28H expression ( Fig. 2c ). As predicted, the most actively dividing T cells are CD28H+ cells for both CD4+ and CD8+ T cells, suggesting that, in response to TCR signal, CD28H-expressing cells are far better proliferators than CD28H− cells ( Supplementary Fig. S7c ). In addition, CD28H− T cells generated by activation exhibited more terminal-differentiated phenotype: they produced less IL-2 but more interferon-γ (IFN-γ), compared with CD28H+ counterparts ( Supplementary Fig. S7d ). Taken together, our data indicated that loss of CD28H in T cell defines as replicative senescence. CD28H delivers a positive costimulatory signal to T cells We first test whether CD28H could function as a possible co-signalling receptor on T cells. Similar to the CD28 family receptors, the intracellular domains of CD28H contain three tyrosines, whose phosphorylation could potentially have a crucial role in signal transduction. We took advantage of the well-known characteristics of agonistic CD28 mAb and constructed various CD28-CD28H chimeric molecules. HEK293T cells were transfected with these chimeric CD28H constructs and then treated with Pervanadate, an irreversible protein-tyrosine phosphatase inhibitor to block endogenous tyrosine phosphorylation. This transfection led to tyrosine phosphorylation of wild-type CD28 and CD28-CD28H chimera but not CD28-CD28H Del mutants ( Fig. 3a ), indicating that tyrosines in the CD28H intracellular domain have the potential to be phosphorylated and therefore to mediate signal transduction. Further studies used site-directed mutagenesis to replace each tyrosine in the intracellular domain of CD28H with phenylalanine. These studies indicated that Y192 and Y222, but not Y197 of CD28H, could potentially be phosphorylated ( Fig. 3b ). Confocal imaging analysis revealed that the CD28H protein was distributed on naive T-cell surface membrane, and seemed to co-localize with CD3. Interestingly, as CD3 redistributed upon T-cell activation, CD28H also became concentrated in the synapse with CD3 without crosslinking of the CD28H receptor ( Fig. 3c ). These results support a possible role for CD28H in the regulation of T-cell receptor signalling events during activation. 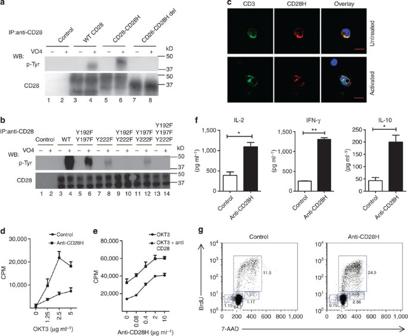Figure 3: CD28H functions as a costimulatory receptor for human T cell. (a,b) Tyrosine phosphorylation of CD28H upon pervanadate treatment. (a) HEK293T cells were transiently transfected with CD28, CD28-CD28H chimera or CD28-CD28H Del plasmid. Cells were incubated in the absence (lane 1, 3, 5, 7) or presence (lane 2, 4, 6, 8) of pervanadate, and analysed for tyrosine phosphorylation. (b) HEK293T cells transfected with wild-type or tyrosine mutants of CD28-CD28H were treated with pervanadate to analyse tyrosine phosphorylation individually. (c) Purified human T cells were incubated in the absence (up) or presence (down) of anti-CD3-coated beads for 1 h, fixed and visualized by confocal microscopy. The co-localization of CD3 (green) and CD28H (red) is presented as overlay (scale bar, 10 μm). (d) Purified naive human CD4+ T cells were stimulated with coated anti-CD28H mAb or control antibody in the presence of titrated anti-CD3.3H-TdR was added during the final 6 h of culture. (e) Proliferation assay of human T cells stimulated with coated anti-CD3 with (●) or without (■) anti-CD28 plus various concentrations of anti-CD28H mAb. (f) Cultured supernatants were collected and cytokine levels were analysed by ELISA. (g) Cultured human T cells were pulsed with BrdU 1 h before collection, and stained with anti-BrdU and 7-AAD. All data are presented as the mean±s.d. and are representative of three experiments. *P<0.05, **P<0.01 (unpaired Student’st-test). IP: immunoprecipitation; WB: western blot. Figure 3: CD28H functions as a costimulatory receptor for human T cell. ( a , b ) Tyrosine phosphorylation of CD28H upon pervanadate treatment. ( a ) HEK293T cells were transiently transfected with CD28, CD28-CD28H chimera or CD28-CD28H Del plasmid. Cells were incubated in the absence (lane 1, 3, 5, 7) or presence (lane 2, 4, 6, 8) of pervanadate, and analysed for tyrosine phosphorylation. ( b ) HEK293T cells transfected with wild-type or tyrosine mutants of CD28-CD28H were treated with pervanadate to analyse tyrosine phosphorylation individually. ( c ) Purified human T cells were incubated in the absence (up) or presence (down) of anti-CD3-coated beads for 1 h, fixed and visualized by confocal microscopy. The co-localization of CD3 (green) and CD28H (red) is presented as overlay (scale bar, 10 μm). ( d ) Purified naive human CD4+ T cells were stimulated with coated anti-CD28H mAb or control antibody in the presence of titrated anti-CD3. 3 H-TdR was added during the final 6 h of culture. ( e ) Proliferation assay of human T cells stimulated with coated anti-CD3 with ( ● ) or without (■) anti-CD28 plus various concentrations of anti-CD28H mAb. ( f ) Cultured supernatants were collected and cytokine levels were analysed by ELISA. ( g ) Cultured human T cells were pulsed with BrdU 1 h before collection, and stained with anti-BrdU and 7-AAD. All data are presented as the mean±s.d. and are representative of three experiments. * P <0.05, ** P <0.01 (unpaired Student’s t -test). IP: immunoprecipitation; WB: western blot. Full size image We next directly tested whether signalling through CD28H could affect T-cell function. We first measured the proliferative response to plated-bound anti-CD3 (OKT3) in the presence of CD28H mAb or control mAb (hamster anti-TNP mAb). As shown in Fig. 3d , CD28H mAb co-immobilized with different concentrations of CD3 mAb greatly enhanced T-cell proliferation compared with the control. The costimulatory effect of CD28H mAb was dose dependent, and its costimulatory effect could be achieved even in the presence of a costimulatory CD28 mAb ( Fig. 3e ). As a result, CD28H-costimulated human T cells produced higher levels of IL-2, as well as IFN-γ and IL-10, than the control mAb ( Fig. 3f ). These results indicate that our CD28H mAb is capable of costimulating T cells in the presence of TCR signalling. Co-signalling molecules could affect T-cell proliferation through promoting the cell cycle or increasing survival [4] , [27] . To distinguish these possibilities, we added 5-bromodeoxyuridine (BrdU) to cultured T cells and evaluated the cell cycle progression and cell death by costaining for BrdU and 7-Aminoactinomycin D (7-AAD), respectively. As shown in Fig. 3g , CD28H mAb treatment greatly increased T cells in S phase compared with the control mAb (24.9% versus 11.5%). However, crosslinking of CD28H did not help to prevent cell death (2.56% versus 1.17%). Thus, our data support the concept that CD28H signalling costimulates T cells through promoting the cell cycle in S phase. We further tested the effect of CD28H mAb in vivo , using a xenograft model of graft-versus-host disease [21] . CD28H mAb was given on days 0 and 2 after human T-cell transfer. This treatment significantly accelerated human T-cell division, as evidenced by CFSE dilution ( Fig. 4a ). In addition, T cells from CD28H mAb-treated mice gained more effector functions. As shown in Fig. 4b , there were significantly more CD4+ T cells expressing membrane-bound CD40L and secreting effector cytokine IFN-γ in CD28H mAb-treated mice, compared with those from control mice. CD28H treatment increased the percentage of CD107a+ CD8+ T cells, as well as IFN− γ-producing cells. Altogether, our results indicate that CD28H costimulation promotes T-cell proliferation and differentiation. 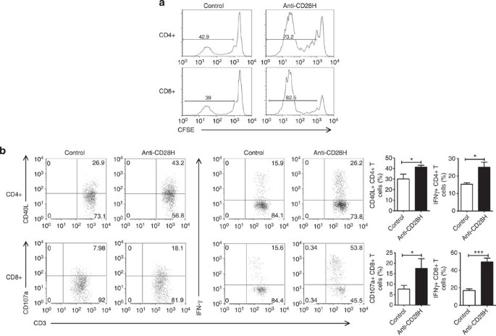Figure 4: Engagement of the CD28H receptor promotes human T-cell responsein vivo. NSG mice transferred with human PBMCs were injected with control or CD28H mAb. Spleen cells were collected on day 6 and were stained for human CD45, CD3 and CD8 to detect transferred human T-cell subsets. (a) Cell division of transferred human T cells. To measure cell division, transferred human PBMCs were labelled with CFSE before transferring. (b) CD40L expression on transferred human CD4+ T cells was detected by flow cytometry right after splenocyte isolation. To detect IFN-γ and/or CD107a-producing cells, splenocytes were restimulatedin vitrofor 5 h. Representative fluorescence-activated cell sorting data were shown on the left, and summarized on the right. All data are presented as the mean±s.d. and are representative of three experiments. *P<0.05, ***P<0.001 (unpaired Student’st-test). Figure 4: Engagement of the CD28H receptor promotes human T-cell response in vivo . NSG mice transferred with human PBMCs were injected with control or CD28H mAb. Spleen cells were collected on day 6 and were stained for human CD45, CD3 and CD8 to detect transferred human T-cell subsets. ( a ) Cell division of transferred human T cells. To measure cell division, transferred human PBMCs were labelled with CFSE before transferring. ( b ) CD40L expression on transferred human CD4+ T cells was detected by flow cytometry right after splenocyte isolation. To detect IFN-γ and/or CD107a-producing cells, splenocytes were restimulated in vitro for 5 h. Representative fluorescence-activated cell sorting data were shown on the left, and summarized on the right. All data are presented as the mean±s.d. and are representative of three experiments. * P <0.05, *** P <0.001 (unpaired Student’s t -test). Full size image Identification of B7-H5 as a ligand for CD28H In an effort to identify its interacting partner, we first tested whether CD28H interacts with any known B7 family member. HEK293T cells were transiently transfected with individual known human B7 ligands and stained with CD28H protein by flow cytometry. We did not find any binding of CD28H protein to HEK293T cells expressing known B7 members ( Supplementary Fig. S8 ). By a high-throughput screening of the receptor array containing over 2,300 transmembrane proteins [28] , we identified a binding candidate and named it B7-H5 ( Fig. 5a ). B7-H5 was previously known as human endogenous retrovirus-H long terminal repeat-associating 2 without an identified function [29] . Interestingly, this molecule has been noted as a new candidate for the B7 family based on a homologue search [30] . By comparing its protein sequence, we demonstrated its homology to other known human B7 ligand members ( Fig. 5b ). Therefore, we assigned the gene a new name B7-H5. B7-H5 has three signature Ig domains (IgV-IgC-IgV) in its extracellular region. Interestingly, the first IgV domain of B7-H5, which presumably contains the receptor-binding domain, has the highest homology with other B7 family members ( Supplementary Fig. S9 ). Notably, mice and rats do not have the ortholog for B7-H5 , which is similar to the CD28H gene. 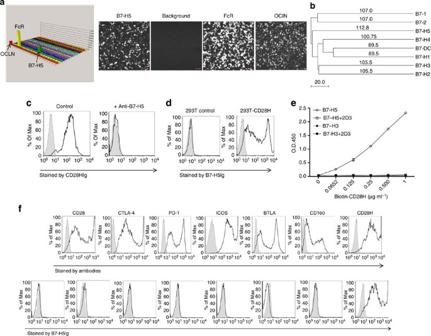Figure 5: Identifying B7-H5 as the ligand for CD28H. (a) Receptor array of a transmembrane protein library with CD28H-mIg fusion protein. Human B7-H5 (HHLA2) was identified as a positive hit besides positive controls, Fc receptor (FcR) and occludin (OCLN) (scale bar, 100 μm). (b) Guide tree analysis of B7-H5 and the known B7 family members. (c,d) Confirmation of the interaction between B7-H5 and CD28H via flow cytometry. (c) B7-H5 transfectant (solid line) or control CHO cells (shaded) was stained with CD28H-Ig, with or without the inclusion of anti-B7-H5 mAb (2D3). (d) HEK293T cells transfected with CD28H or control plasmid were stained with B7-H5 fusion protein. (e) Coated B7-H5 or control protein (B7-H3) was preincubated with or without B7-H5 mAb (clone 2D3), and the ELISA signal was later carried out with the inclusion of biotin-labelled CD28H. (f) HEK293T cells were transfected with individual B7 receptor family members and stained with B7-H5 fusion protein. The expression of each B7 receptor family member was verified by a mAb specific for the respective molecules. Figure 5: Identifying B7-H5 as the ligand for CD28H. ( a ) Receptor array of a transmembrane protein library with CD28H-mIg fusion protein. Human B7-H5 (HHLA2) was identified as a positive hit besides positive controls, Fc receptor (FcR) and occludin (OCLN) (scale bar, 100 μm). ( b ) Guide tree analysis of B7-H5 and the known B7 family members. ( c , d ) Confirmation of the interaction between B7-H5 and CD28H via flow cytometry. ( c ) B7-H5 transfectant (solid line) or control CHO cells (shaded) was stained with CD28H-Ig, with or without the inclusion of anti-B7-H5 mAb (2D3). ( d ) HEK293T cells transfected with CD28H or control plasmid were stained with B7-H5 fusion protein. ( e ) Coated B7-H5 or control protein (B7-H3) was preincubated with or without B7-H5 mAb (clone 2D3), and the ELISA signal was later carried out with the inclusion of biotin-labelled CD28H. ( f ) HEK293T cells were transfected with individual B7 receptor family members and stained with B7-H5 fusion protein. The expression of each B7 receptor family member was verified by a mAb specific for the respective molecules. Full size image To validate the interaction between B7-H5 and CD28H, we generated mAbs to human B7-H5 by immunizing BALB/c mice with a B7-H5-Ig fusion protein. One B7-H5 mAb, clone 2D3, specifically bound B7-H5-transfected cells but not mock-transfected cells ( Supplementary Fig. S2b ). The receptor array screening results were confirmed by flow cytometry, as the CD28H-Ig fusion protein specifically bound to stable B7-H5 CHO transfectants but not to control CHO cells ( Fig. 5c left). Importantly, inclusion of 2D3 was able to completely block this interaction ( Fig. 5c right). Similarly, we transiently transfected HEK293T cells with CD28H and stained with B7-H5-Ig. B7-H5-Ig bound strongly to the HEK293T cells transfected with CD28H, but not to the control plasmid, further suggesting that B7-H5 binds specifically to CD28H ( Fig. 5d ). The direct interaction between B7-H5 and CD28H was also verified by enzyme-linked immunosorbent assay (ELISA). As shown in Fig. 5e , biotin-labelled CD28H protein directly interacted with immobilized B7-H5, but not B7-H3 protein, and this binding could be completely blocked when the plate was preincubated with 2D3. We also excluded the possibility that B7-H5 interacts with other CD28 family members. As shown in Fig. 5f , B7-H5-Ig did not bind to any known CD28 family receptors other than CD28H. Furthermore, the receptor array screening using B7-H5-Ig as the bait identified CD28H as the only binding partner for B7-H5 in our Array library ( Supplementary Fig. S10 ). Therefore, the B7-H5/CD28H interaction represents a new independent pathway related to the classic B7/CD28 family. The expression pattern of B7-H5 Early study by northern blotting indicated that B7-H5 mRNA was enriched in peripheral organs [29] . By PCR, we detected abundant levels of B7-H5 mRNA in testis, colon, lung, kidney and pancreas while its transcript level was low in the small intestine, liver and skeletal muscle ( Fig. 6a ). In immune cells, the B7-H5 transcript was undetectable in T cells, while B cells, dendritic cells and macrophages contained abundant B7-H5 mRNA ( Fig. 6b ). No cell surface B7-H5 expression was detected on T, B, NK cells or monocytes freshly isolated from human PBMCs by 2D3 staining ( Fig. 6c ). However, substantial cell surface B7-H5 could be detected on monocyte-derived macrophages and could be further upregulated by poly (I:C) ( Fig. 6d ). Monocyte-derived dendritic cells expressed minimal levels of B7-H5 protein; however, incubation of dendritic cells with IFN-γ, poly I:C or heat-killed Listeria monocytogenes was capable of inducing B7-H5 expression while lipopolysaccharide had marginal effect ( Fig. 6d ). Our data suggest that B7-H5 is largely an inducible molecule on APCs responding to inflammation. 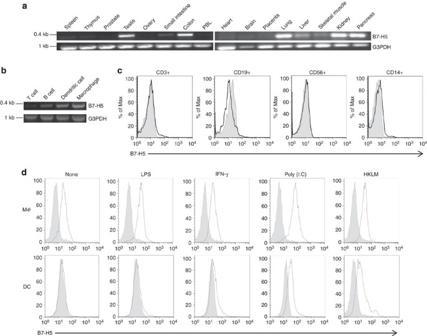Figure 6: B7-H5 expression. Distribution of the B7-H5 transcript. B7-H5 mRNA in different human tissues (a) or immune cell types (b) was detected by PCR. (c) Surface B7-H5 expression on different cell types from freshly isolated hPBMCs. (d) Macrophages or dendritic cells derived from purified human monocytes were treated with lipopolysaccharide (LPS), IFN-γ, poly I:C or heat-killed Listeria monocytogenes (HKLM), and stained with B7-H5 mAb (solid line) or isotype control (shaded). Figure 6: B7-H5 expression. Distribution of the B7-H5 transcript. B7-H5 mRNA in different human tissues ( a ) or immune cell types ( b ) was detected by PCR. ( c ) Surface B7-H5 expression on different cell types from freshly isolated hPBMCs. ( d ) Macrophages or dendritic cells derived from purified human monocytes were treated with lipopolysaccharide (LPS), IFN-γ, poly I:C or heat-killed Listeria monocytogenes (HKLM), and stained with B7-H5 mAb (solid line) or isotype control (shaded). Full size image B7-H5/CD28H interaction costimulates human T-cell responses To test the potential function of B7-H5 on T-cell activation, we incubated purified CD4+ human T cells with plate-coated B7-H5-Ig in the presence of anti-CD3 mAb to mimic TCR ligation. Similar to B7-1, immobilized B7-H5-Ig strongly promoted CD4+ T-cell proliferation. B7-H5 had a costimulatory role because the B7-H5-Ig did not enhance T-cell response in the absence of the anti-CD3 mAb ( Fig. 7a ). Furthermore, B7-H5 increased a variety of cytokine production, including IL-2, IFN-γ, tumour-necrosis factor and IL-10 ( Fig. 7b ). Addition of CD28H-Ig or a B7-H5 mAb (2D3) significantly reduced the costimulatory effect of B7-H5 ( Fig. 7c ), indicating that B7-H5 promotes the T-cell response through CD28H on T cells. 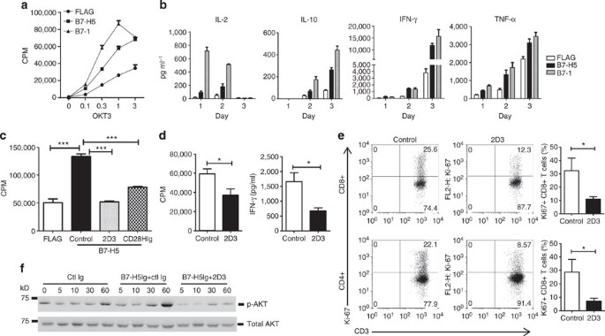Figure 7: B7-H5 engagement costimulates human T cells through CD28H. (a,b) Purified human CD4+ T cells were negatively selected and stimulated with OKT3 together with coated B7-H5, the control protein FLAG, and B7-1 fusion protein. (a)3HTdR was added during the final 6 h of culture. (b) Cultured supernatants were collected and cytokines were measured at different time points. (c) Human CD4 T cells were stimulated with coated B7-H5 or control protein. B7-H5 mAb or CD28H fusion protein was included during cell culture. (d) Human CD4+ T cells were cultured with irradiated macrophages derived from monocytes of another donor in the presence of anti-B7-H5 or control antibody. Proliferation and IFN-γ production were measured 5 days after culture. (e) Humanized NSG mice were challenged with allogeneic human macrophages. At the same day, each mouse was inoculated with control or anti-B7-H5 (clone 2D3) mAb. On day 7, splenocytes were collected and stained for human CD3 and CD8, and Ki-67. Representative fluorescence-activated cell sorting data were shown on the left, and summarized on the right. (f) AKT phosphorylation upon B7-H5 stimulation. All data are presented as the mean±s.d. and are representative of three experiments. *P<0.05, ***P<0.001 (unpaired Student’st-test). CPM: counts per minute. Figure 7: B7-H5 engagement costimulates human T cells through CD28H. ( a , b ) Purified human CD4+ T cells were negatively selected and stimulated with OKT3 together with coated B7-H5, the control protein FLAG, and B7-1 fusion protein. ( a ) 3 HTdR was added during the final 6 h of culture. ( b ) Cultured supernatants were collected and cytokines were measured at different time points. ( c ) Human CD4 T cells were stimulated with coated B7-H5 or control protein. B7-H5 mAb or CD28H fusion protein was included during cell culture. ( d ) Human CD4+ T cells were cultured with irradiated macrophages derived from monocytes of another donor in the presence of anti-B7-H5 or control antibody. Proliferation and IFN-γ production were measured 5 days after culture. ( e ) Humanized NSG mice were challenged with allogeneic human macrophages. At the same day, each mouse was inoculated with control or anti-B7-H5 (clone 2D3) mAb. On day 7, splenocytes were collected and stained for human CD3 and CD8, and Ki-67. Representative fluorescence-activated cell sorting data were shown on the left, and summarized on the right. ( f ) AKT phosphorylation upon B7-H5 stimulation. All data are presented as the mean±s.d. and are representative of three experiments. * P <0.05, *** P <0.001 (unpaired Student’s t -test). CPM: counts per minute. Full size image To further evaluate the function of endogenous B7-H5/CD28H interaction on the T-cell response, we stimulated human T cells with preactivated allogeneic macrophages. The inclusion of 2D3 significantly reduced the allogeneic T-cell proliferation ( Fig. 7d left) and IFN-γ secretion ( Fig. 7d right). We further examined whether blockade of the B7-H5/CD28H pathway could alleviate allogeneic T-cell responses in vivo . Humanized NSG mice were challenged with allogeneic macrophages intraperitoneally. As shown in Fig. 7e , administration of 2D3 significantly inhibited human T-cell proliferation, based on Ki-67 staining. Taken together, our results support that endogenous B7-H5/CD28H interaction has an important role in allogeneic T-cell response. B7-CD28 costimulation is known to activate the phosphoinositide 3-kinase– and serine–threonine kinase AKT-dependent signalling cascade and promote cellular proliferation and T-cell activation [31] , [32] . We activated human T cells with immobilized anti-CD3 and B7-H5 or control Ig proteins. As shown in Fig. 7f , simultaneous crosslinking of TCR and B7-H5 induced AKT phosphorylation 30 min after stimulation, while TCR crosslinking alone induced minimal AKT phosphorylation. Importantly, inclusion of 2D3 prevented AKT activation, indicating that B7-H5 costimulation presumably utilizes the AKT pathway to promote T-cell response. CD28H ligation regulates antigen-specific T-cell responses We further evaluated the effects of CD28H-B7-H5 pathway in an antigen-specific T-cell response. Purified human CD4+ T cells were labelled with CFSE, and cultured with autologous monocyte-derived dendritic cells preincubated with tetanus toxoid (TT). TT-specific T-cell proliferation was strongly augmented when agonistic CD28H mAb was included in the culture to amplify CD28H signal on T cells ( Fig. 8a ). Inclusion of CTLA4-Ig, a fusion protein blocking B7-CD28 interactions, at the beginning of cell culture greatly inhibited T-cell proliferation, even in the presence of agonistic CD28H mAb. Our results indicate that CD28H costimulation may be dependent on endogenous B7-CD28 interaction. We also noted a substantial enhancement of cytokine production by CD28H agonistic antibody, including IFN-γ, IL-5, IL-10, tumour-necrosis factor-α and IL-17 ( Fig. 8b ). 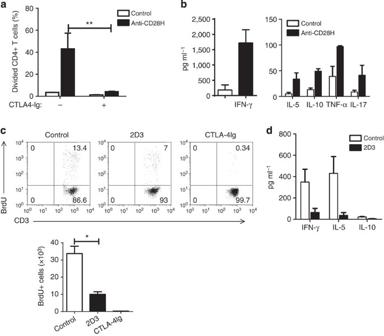Figure 8: The effect of B7-H5/CD28H interaction in TT-specific T-cell response. (a,b) Human PBMCs were labelled with CFSE, and were co-cultured with autologous dendritic cells preincubated with TT. Control or CD28H mAb were included in the beginning of culture in the presence or absence of CTLA4-Ig. (a) The proliferation of TT-specific CD4+ T cells was determined by CFSE dilution of the human CD3 and CD4 double-positive cells. (b) Supernatant from the culture was analysed for cytokine level as indicated. (c,d) NSG mice reconstituted with human PBMCs, and autologous dendritic cells were immunized with TT vaccine. At the same day, mice were treated with control Ig, 2D3 (anti-B7-H5 mAb) or CTLA4-Ig. (c) Seven days later, cells in the peritoneal cavity were harvested, and restimulated with TT antigen. T-cell division was analysed by BrdU incorporation. (d) Cytokines in the culture supernatant were examined by a human Th1/Th2 CBA kit. All data are presented as the mean±s.d. and are representative of two experiments. *P<0.05, **P<0.01 (unpaired Student’st-test). Figure 8: The effect of B7-H5/CD28H interaction in TT-specific T-cell response. ( a , b ) Human PBMCs were labelled with CFSE, and were co-cultured with autologous dendritic cells preincubated with TT. Control or CD28H mAb were included in the beginning of culture in the presence or absence of CTLA4-Ig. ( a ) The proliferation of TT-specific CD4+ T cells was determined by CFSE dilution of the human CD3 and CD4 double-positive cells. ( b ) Supernatant from the culture was analysed for cytokine level as indicated. ( c , d ) NSG mice reconstituted with human PBMCs, and autologous dendritic cells were immunized with TT vaccine. At the same day, mice were treated with control Ig, 2D3 (anti-B7-H5 mAb) or CTLA4-Ig. ( c ) Seven days later, cells in the peritoneal cavity were harvested, and restimulated with TT antigen. T-cell division was analysed by BrdU incorporation. ( d ) Cytokines in the culture supernatant were examined by a human Th1/Th2 CBA kit. All data are presented as the mean±s.d. and are representative of two experiments. * P <0.05, ** P <0.01 (unpaired Student’s t -test). Full size image We also evaluated the role of this costimulatory interaction on TT-specific T-cell response in vivo . In this model, NSG mice were transferred with human PBMCs together with autologous monocyte-derived dendritic cells, and were immunized with TT vaccine. Endogenous B7-H5/CD28H interaction appears to be important for the recall of TT-specific memory T cells because injection of the mice with B7-H5-blocking mAb 2D3 significantly inhibited TT vaccine-elicited T-cell proliferation, as indicated by BrdU incorporation ( Fig. 8c ). Inoculation of CTLA-4Ig, a positive control, completely abrogated the TT vaccine-induced T-cell proliferation. As a result, cytokines in the culture supernatant including IFN-γ, IL-5 and IL-10 were all substantially reduced by the 2D3 mAb ( Fig. 8d ). Taken together, our studies supported that the B7-H5/CD28H interaction has an important role in the recall of memory T cells. In this study we describe a new cell surface molecular interaction between CD28H and B7-H5 with costimulatory functions for T cells. Similar to parental CD28 molecule, CD28H is constitutively expressed in naive T and NK cells, and transmits a costimulatory signal to T cells through AKT pathway. CD28H accumulates at the immunological synapse upon T-cell activation without ligand binding, a feature shared by CD28 (ref. 33 ). In addition, CD28H appears to be a pan-T-cell activator and costimulates T cells without bias to different subsets. It has been shown that repetitive stimulation of human CD4+ T cells will lead to permanent loss of CD28 on the cell surface, which is associated with T-cell senescence [34] . Similarly, repeated stimulations of human T cells eliminate CD28H expression, and the phenotypes of these CD28H− cells are similar to those ageing T cells. However, several major features distinguish this pathway from the classic B7/CD28 pathway. In contrast to B7-1 and B7-2, which are limited on professional APCs, B7-H5 could be found abundantly in peripheral tissues. In the context of these findings, the B7-H5/CD28H interaction appears to be critical for the costimulation of newly generated effector or effector/memory T cells in peripheral tissues in addition to lymphoid organs. Another important difference is that the B7-H5/CD28H interaction is not present in mice and rats. It is worthwhile to note that a recently identified B7-H2/CD28 interaction is also not found in mice [28] . Thus, these findings may warrant reassessment of the B7-CD28 costimulatory system in humans. Unlike other known B7 members, the extracellular domain of B7-H5 contains three Ig domains rather than the two Ig domains, with an exception of two duplicated IgV-IgC in human B7-H3 (ref. 35 ). Its counter receptor, CD28H, also an Ig superfamily member, shares structural similarity with other CD28 family molecules. Neither B7-H5 nor CD28H bound other known B7 receptors or ligands, respectively. In addition, CD28H does not bind B7-H5− APCs, such as monocytes or immature dendritic cells ( Supplementary Fig. S11 ). Over 20 human tumour lines we examined, CD28H only bound three B7-H5+ human cell lines. Inclusion of a B7-H5-blocking mAb completely abolished these bindings ( Supplementary Table S1 and Supplementary Fig. S11 ). All these suggest that B7-H5/CD28H interaction represents an independent B7 pathway. CD28H is constitutively expressed on all naive human T cells. However, a significant percentage of effector/memory T cells from human PBMCs lost CD28H expression. Though B7-H5 is expressed at relatively low levels on resting dendritic cells and macrophages, it could be upregulated in response to a variety of inflammatory stimuli. These data implicate that, in the presence of inflammation, CD28H could provide a positive signal during naive T-cell priming. However, in contrast to the restricted expression of B7-1 and B7-2 to professional APCs, B7-H5 was abundantly found in peripheral non-hematopoietic organs, implying a preferential role for B7-H5 in peripheral tissues. As effector memory T cells reside in extra-lymphoid sites and provide fast-responding immune surveillance against infections and tumours, the presence of B7-H5 could provide a better immune microenvironment for the recall response of memory T cells [36] , [37] , [38] . However, excessive T-cell response could also be destructive during autoimmune diseases and chronic infections. Under these conditions, the gradual loss of CD28H expression upon exposure to antigens would provide a self-protective mechanism to restrain the T-cell response. Taken together, our results describe a new costimulatory pathway, which is independent of other known B7 family members. Its potential involvement in human diseases, however, has yet to be elucidated. It is valuable to further investigate the B7-H5/CD28H pathway in patients with autoimmune diseases or cancer, which would ultimately reveal new potential therapeutic interventions. Plasmids and fusion proteins The plasmids for B7-H5 and CD28H full-length cDNA were purchased from the Open Biosystems Inc. (Huntsville, AL). They were cloned into the pcDNA3.1(−) vector by PCR. The extracellular domains of B7-H5 and CD28H were cloned and fused into pmIgV expression vectors containing the constant region of mouse IgG2a [39] . Fusion proteins were expressed by transiently transfecting HEK293T cells using the calcium phosphate precipitation method, and fusion proteins were purified using a Protein A Sepharose column according to the manufacturer’s instructions (GE Healthcare). To enhance the secretion of fusion protein, the native signal peptide of B7-H5 was replaced with the preprotrypsin signal peptide derived from the pCMV FLAG vector (Sigma, MO). Antibodies Mouse anti-human B7-H5 mAb (clone 2D3) was generated from a hybridoma derived from the fusion of SP2 myeloma with B cells from a mouse immunized with human B7-H5-Ig. Hamster anti-human CD28H mAb (clone 4–5) was generated from a hybridoma derived by fusion of SP2 myeloma with B cells from an Armenian hamster immunized with human CD28H-Ig [40] . Hybridomas was cultured in RPMI with 10% fetal bovine serum. Antibodies in supernatant were purified by Hitrap protein G affinity column (GE Healthcare). Anti-human Ig and anti-mouse Ig FMAT blue antibody were purchased from Applied Biosystems (Foster City, CA). Control hamster IgG and hamster anti-mouse TNP were purchased from eBioscience. All other antibodies used in flow cytometry were purchased from BD Bioscience (San Jose, CA), eBioscience or Biolegend. Rabbit anti-total AKT and anti-phospho-AKT (Ser473) were purchased from Cell Signaling (Danvers, MA). Screening of the receptor array Plasmids containing over 2,300 human transmembrane genes were placed individually into several 384-well plates at 60 ng per well. Lipofectamine 2000 was added to each well and mixed with plasmids for 30 min. Ten thousand 293T cells were added subsequently to each well to perform transient transfection. Eight hours after transfection, 50 ng human CD28H-Ig or B7-H5-Ig and 50 ng anti-mouse Ig FMAT blue secondary antibody were added into each well. The plates were read 24 h after transfection by the Applied Biosystems 8,200 cellular detection system and analysed by CDS 8,200 software. Each plate has a well containing the Fc receptor as an internal positive control for transfection. Chimeras and tyrosine mutants The CD28-CD28H chimera, which contains the extracellular domains of CD28 but the transmembrane and intracellular domains from CD28H, was generated by PCR. The CD28-CD28H del mutant with deleted intracellular domains was generated by PCR using CD28-CD28H as the template. Mutants for the three tyrosines (Y192, Y197 and Y222) in CD28H intracellular domain were made by changing respective tyrosine (Y) to phenylalanine (F). Double and triple tyrosine-to-phenylalanine mutations were further generated by using one primer pair to PCR with a single or double tyrosine-mutated template. HEK293T cells transfected with individual plasmid were incubated in the presence or absence of 100 μM pervanadate for 10 min. Cells were lysed for 30 min in lysis buffer at 4 °C and centrifuged at 14,000 g for 10 min. The supernatant was immunoprecipitated with 1 μg CD28 mAb and 20 μl of protein G-magnetic beads (Invitrogen). After being washed with lysis buffer three times, the pellets were boiled for 10 min with 3 × SDS–polyacrylamide gel electrophoresis loading buffer and resolved on 10% polyacrylamide gels. After being transferred to nitrocellulose, blots were analysed for phosphotyrosine using 4G10 (Millipore) or CD28 using biotinlated-anti-CD28 (R&D system). Immunohistochemistry staining and flow cytometry analysis Immunohistochemistry for CD28H was performed with CD28H mAb (clone 4–5) at a concentration of 5 μg ml −1 according to a standard protocol [41] . For cell surface staining and analysis by flow cytometry, cells were incubated with the indicated mAb for 30 min at 4 °C, washed with buffer and analysed. For intracellular cytokine analysis, T cells were restimulated with phorbol myristate acetate plus ionomysin in the presence of brefeldin A. The cells were then stained with indicated mAb to cell surface molecules, cytokine antibodies or control for 30 min at 4 °C, fixed and permeabilized before analysis. For CD107a staining, PE-labelled CD107a and isotype control antibody were added during the culture. T-cell proliferation assay Human PBMCs from healthy donors were purchased from Research Blood Components (Brighton, MA). OKT mAb (anti-human CD3) was precoated in the 96-well plates at the indicated concentrations. B7-H5.Ig, anti-CD28H, B7-1 or control Ig at 5 μg ml −1 were also immobilized in the wells. Human peripheral blood T cells were negatively selected and purified by a human pan-T-cell selection kit or naive human CD4 T-cell selection kit (Miltenyi Biotec, Auburn, CA). T cells were added into each well at 2.5–3 × 10 5 per well and cultured for 3 days. In some experiments, costimulatory anti-human CD28 was added at the beginning of the culture. 3 H-thymidine (TdR) was added during the final 6 h of culture. 3 H-TdR incorporation was counted with a MicroBeta Trilux liquid scintillation counter (Wallac). Cytokine measurement Supernatant from the T-cell costimulation assays were collected. Human IFN-γ, IL-2 and IL-10 were detected by ELISA (BD PharMingen or eBioscience). In some experiments, cytokine levels in the supernatant were analysed using a BD Cytometric Bead Array (CBA) Kit, according to the manufacturer’s instructions. Xenogeneic graft-versus-host disease model Female NSG mice (Jackson Lab) were intraperitoneally transferred with 15–20 million human PBMCs or 10 million purified naive CD4+ human T cells. On days 0 and 2, each mouse was inoculated peritoneally with 300 μg control or CD28H mAb. Six days after transfer, splenocytes were collected. Human T cells were detected by staining for human CD45, CD3 and CD8. Splenocytes were restimulated in vitro with phorbol myristate acetate plus ionomycin to detect IFN-γ or CD107a-producing cells. To monitor cell division, hPBMCs were labelled with CFSE before transfer. All mouse protocols were in accordance with NIH guidelines and were approved by the Animal Care and Use Committee of the Johns Hopkins University School of Medicine and Yale University School of Medicine. Allogeneic T-cell responses in a humanized mouse model Human CD133 + CD34 + cells were purified from fresh umbilical cord blood and were transferred into sub-lethally irradiated neonates NOD - SCID Il2rg −/ − (NSG) mice by intracardiac injection within the first 48 h after birth. Reconstitution of the human immune system in the NSG mice was confirmed by examining human CD45+ cells in the mouse peripheral blood by flow cytometry 12 weeks post engraftment. Mice were adoptively transferred with two million allogeneic macrophages. At the same day, each mouse was inoculated with 500 μg control or anti-B7-H5 (clone 2D3) mAb. Seven days later, mice were killed and splenocytes were collected. Human T-cell subsets were detected by staining for human CD3 and CD8. Cellular proliferation was examined by intracellular staining of Ki-67. Tetanus toxoid-specific human T-cell response For in vitro TT stimulation, dendritic cells were incubated with 2 μg ml −1 TT (List Biological Laboratories) overnight. After washed with culture medium, DCs were co-cultured with CFSE-labelled synergistic human PBMCs at 1:10 ratio for 7–10 days. Antibodies and fusion proteins were added from the beginning of culture. Cell division of human CD4+ T cells was examined by fluorescence-activated cell sorting for CFSE dilution. At the same time, cytokines in supernatant from the culture was checked by a human Th1/Th2/Th17 CBA Kit (BD Bioscience). To study TT immunization in vivo , we intraperitoneally transferred 6–8 million human PBMCs along with 0.6 million synergistic dendritic cells into each NSG mouse. At the same time, each mouse was immunized with 1/30 dose of TENIVAC (0.5 ml, Sanofi Pasteur). Mice were divided into three groups, and were treated with 250 μg control Ig, 2D3 or CTLA4-Ig respectively. Seven days later, cells in the peritoneal were washed out by cold PBS, counted and restimulated with synergistic DCs preincubated with TT. BrdU was added from the beginning to record T-cell proliferation. On day 7, supernatant was collected to check cytokine level, and cells were collected to study T-cell division by BrdU incorporation. T-cell lysate preparation and immunoblot Purified human CD4 + T cells from healthy donors were activated with 1 μg ml −1 immobilized anti-CD3 (OKT3) for 3 days, and rested for another 3 days in the presence of 50 IU ml −1 rhIL-2. T cells were subsequently collected and added into 96-well plates precoated with 0.01 μg ml −1 anti-CD3 plus 10 μg ml −1 B7-H5-Ig or control Ig proteins. In some wells, anti-B7-H5 (2D3) or control Ig were included in the culture. Cells were collected at different time points as indicated. Cell lysates were prepared. Hundred microgram of total protein per sample was loaded and separated by 12% SDS–polyacrylamide gel electrophoresis. The amount of phosphorylated AKT protein was determined by immunoblotting with Ser473 phospho-specific AKT antibodies. Membrane was subsequently striped and reprobed with antibodies against total AKT. Statistical analysis Student’s t -test was used for statistical analysis, and P -values reflect comparison with the control sample. P -values less than 0.05 were considered statistically significant. *The error bars in figures represent s.d. How to cite this article: Zhu, Y. et al. B7-H5 costimulates human T cells via CD28H. Nat. Commun. 4:2043 doi: 10.1038/ncomms3043 (2013).